Atomistic insight into viscosity and density of silicate melts under pressure A defining characteristic of silicate melts is the degree of polymerization (tetrahedral connectivity), which dictates viscosity and affects compressibility. While viscosity of depolymerized silicate melts increases with pressure consistent with the free-volume theory, isothermal viscosity of polymerized melts decreases with pressure up to ~3–5 GPa, above which it turns over to normal (positive) pressure dependence. Here we show that the viscosity turnover in polymerized liquids corresponds to the tetrahedral packing limit, below which the structure is compressed through tightening of the inter-tetrahedral bond angle, resulting in high compressibility, continual breakup of tetrahedral connectivity and viscosity decrease with increasing pressure. Above the turnover pressure, silicon and aluminium coordination increases to allow further packing, with increasing viscosity and density. These structural responses prescribe the distribution of melt viscosity and density with depth and play an important role in magma transport in terrestrial planetary interiors. Understanding the structural response of silicate melts to pressure and composition is crucial in earth and planetary sciences, as the differentiation of chemical species within planetary interiors is primarily controlled by melting and crystallization processes, which are intimately linked to evolution histories and thermal states of the planets [1] , [2] , [3] . Quenching of pressurized oxide melts may also produce new materials, such as densified glasses with novel and tailored properties [4] , [5] , [6] . The degree of polymerization, a key to understanding tetrahedral oxide melts such as silicates, is characterized by the ratio of non-bridging oxygen (NBO) per tetrahedron, NBO/T (where T represents tetrahedrally coordinated cations Si, Al, Ti and so on, and an NBO is an oxygen bonded to only one T atom) [7] . At ambient pressure, since almost all the oxygen atoms form either non-bridging (T–O) or bridging (T–O–T) bonds, NBO/T can be obtained simply from the ratio of O/T present in a given system with good accuracy (NBO≈2 × O–4 × T) [7] . In fully polymerized melts with NBO/T≈0, essentially all the oxygen atoms in each TO 4 tetrahedron are linked to adjacent tetrahedra, forming three-dimensional (3D) networks with high viscosities at ambient pressure. Depolymerized melts, with NBO/T≥2, however, have lower tetrahedral connectivity and lower viscosity at 1 atm (ref. 8 ). 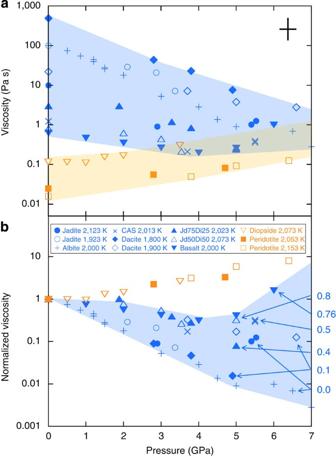Figure 1: Pressure-viscosity behaviour of polymerized (NBO/T<1) and depolymerized (NBO/T=2) silicate melts. (a) Viscosities of polymerized melts (blue symbols and shaded area), generally with higher values at 1 atm, exhibit negative pressure dependence at low pressures. The range of viscosity variation decreases with pressure (blue shaded area). Reversal in pressure dependence is observed in many polymerized melts. For depolymerized melts, viscosities generally increase with pressure (orange symbols and shaded area). Typical experimental uncertainties are given. (b) Normalized viscosities with respect to their 1 atm values. Pressure turnover is more clearly seen for the polymerized melts (blue symbols and shaded area). Approximate values of NBO/T for the polymerized melts are given on the right side of the figure. Magnitude of the viscosity decrease appears to be inversely correlated to the NBO/T ratio and temperature. Normalized viscosities of depolymerized melts (orange symbols, with NBO/T≈2) fall in a very narrow range and are not shaded. Figure 1 and Table 1 summarize experimentally measured viscosities of anhydrous silicate melts at high pressure [9] , [10] , [11] , [12] , [13] , [14] , [15] , [16] , [17] . Melts containing volatiles such as water and CO 2 are not considered here. The response of viscosities to pressure is strikingly distinct between polymerized (NBO/T<1) and depolymerized (NBO/T≥2) melts [17] : while viscosities of depolymerized melts such as diopside (Di; CaMgSi 2 O 6 , NBO/T≈2) [18] increase monotonically (a normal behaviour consistent with the free-volume theory), those of polymerized melts such as jadeite [9] (Jd; NaAlSi 2 O 6 , NBO/T≈0) and basalt [16] (NBO/T≈0.7) first decrease with increasing pressure (abnormal). In addition to this abnormal negative pressure dependence, most of the polymerized melts also exhibit a viscosity minimum along an isotherm, though in some cases the turnover is not observed within the experimental pressure range. Figure 1: Pressure-viscosity behaviour of polymerized (NBO/T<1) and depolymerized (NBO/T=2) silicate melts. ( a ) Viscosities of polymerized melts (blue symbols and shaded area), generally with higher values at 1 atm, exhibit negative pressure dependence at low pressures. The range of viscosity variation decreases with pressure (blue shaded area). Reversal in pressure dependence is observed in many polymerized melts. For depolymerized melts, viscosities generally increase with pressure (orange symbols and shaded area). Typical experimental uncertainties are given. ( b ) Normalized viscosities with respect to their 1 atm values. Pressure turnover is more clearly seen for the polymerized melts (blue symbols and shaded area). Approximate values of NBO/T for the polymerized melts are given on the right side of the figure. Magnitude of the viscosity decrease appears to be inversely correlated to the NBO/T ratio and temperature. Normalized viscosities of depolymerized melts (orange symbols, with NBO/T≈2) fall in a very narrow range and are not shaded. Full size image Table 1 Experimentally determined pressure dependence of viscosity along various isotherms (for polymerized silicate melts with NBO/T<1). Full size table There are, however, some discrepancies to this general behaviour. For example, a decrease in viscosity was reported in Di melt (depolymerized) between 8.5 and 13 GPa (ref. 19 ) and attributed to increased Si–O coordination. Molecular dynamics (MD) analysis [20] , however, showed only a monotonic increase in viscosity of Di melt up to 20 GPa. Part of the discrepancy may be attributed to the difficulty in accurately determining viscosities at high pressure. One of the best high-pressure techniques developed thus far is the falling-sphere viscometry [21] , which yields viscosity data with typical uncertainties of ~0.5 decade in units of Pa s. Pressure and temperature are also difficult to measure accurately under molten conditions. The general trend in Fig. 1 is supported by measurements on oxygen self-diffusivity, D ( O ), which is related to viscosity of the melt, η , by the Eyring relation [22] , η= ( k B T )/( D ( O ) λ ), where k B is Boltzmann constant, T temperature in K and λ the ‘jump distance’ for self-diffusion. Numerous studies report D ( O ) maxima in polymerized silicate melts along isothermal compression, for example, ~5 GPa for albite [23] and dacite [24] , and ~8 GPa for Na 3 AlSi 7 O 17 (ref. 23 ), implying a reversal in pressure dependence. MD simulations on SiO 2 melt (NBO/T=0) also reveal maxima in O and Si self-diffusivity on compression [5] , [25] . More than 200 ‘zero-pressure’ (that is, 0.1 MPa) bulk moduli (K T0 ) data points of anhydrous liquid silicates in the Ca–Mg–Fe–Na–K–Al–Si–O system, determined by the ultrasonic technique [26] and linear mixing models for bulk modulus [27] , [28] , fall in a narrow range of 14–25 GPa at temperatures from 1,573 to 1,800 K ( Fig. 2a ). Although the 17 ultrasonic data points [26] hint on a positive dependence on NBO/T, 185 values from the equation of state fits [27] show no clear trend. Available pressure derivatives (K T0 ′), in contrast, decrease systematically with increasing SiO 2 content [28] . When these K T0 ′ data are plotted against NBO/T, a clear positive trend emerges ( Fig. 2b ). This suggests that polymerized liquids are generally more compressible than depolymerized liquids with increasing pressure. 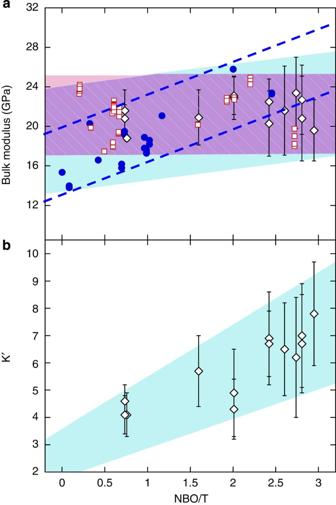Figure 2: Correlations of ambient pressure KT0and KT0′ of silicate liquids with NBO/T. (a) Relaxed bulk moduli according to the ultrasonic technique26at 1,673±100 K (solid circles; plus anorthite melt at 1,833 K—solid hexagon) and thermal equation of state fits to literature data between 1,573 and 1,800 K (open squares—ref.27; open diamonds—ref.28) in the system Ca–Mg–Na–K–Al–Si–O (excluding (Na,K)xSiyOzmelts from the database in ref.27). Although data from ref.26display a positive correlation (shown by the two dashed lines), the 185 points from refs27,28show no correlation (the purple, horizontal shaded band). (b) KT0′ of natural silicate liquids reported in ref.28, plotted against NBO/T, showing a positive correlation. In both (aandb) NBO/T ratios are calculated based on compositions of the liquids according to NBO=2 × O—4 × T. Al is assumed to be in the tetrahedral site and Fe is assumed to be Fe2+. Figure 2: Correlations of ambient pressure K T0 and K T0 ′ of silicate liquids with NBO/T. ( a ) Relaxed bulk moduli according to the ultrasonic technique [26] at 1,673±100 K (solid circles; plus anorthite melt at 1,833 K—solid hexagon) and thermal equation of state fits to literature data between 1,573 and 1,800 K (open squares—ref. 27 ; open diamonds—ref. 28 ) in the system Ca–Mg–Na–K–Al–Si–O (excluding (Na,K) x Si y O z melts from the database in ref. 27 ). Although data from ref. 26 display a positive correlation (shown by the two dashed lines), the 185 points from refs 27 , 28 show no correlation (the purple, horizontal shaded band). ( b ) K T0 ′ of natural silicate liquids reported in ref. 28 , plotted against NBO/T, showing a positive correlation. In both ( a and b ) NBO/T ratios are calculated based on compositions of the liquids according to NBO=2 × O—4 × T. Al is assumed to be in the tetrahedral site and Fe is assumed to be Fe 2+ . Full size image The above systematics are consistent with the rigidity percolation theory [29] , which predicts that 2.4 connections are required between each structural unit to form a fully continuous 3D network. For tetrahedral random networks, this means that when NBO/T≥1.6, there are too few tetrahedron–tetrahedron connections to form fully continuous 3D networks [30] . Unlike chalcogenide systems, here percolation (or rigidity) is applied to inter-tetrahedral bonds instead of interatomic bonds, as TO 4 are considered to act like fixed units in silicate liquids. This physical description is valid only at low pressures. Structural analyses on super-cooled silicate liquids show that with increasing pressure, oxygen tri-clusters (O connected to three T atoms) and coordinations higher than tetrahedral come into play [31] ; structures of the melts can no longer be represented by simple corner-sharing tetrahedral networks. In the present study, we conduct structural analyses on melts along the Jd–Di join at high pressure. These compositions are chosen because viscosities of melts along this join, which represent a large range of NBO/T, have been well studied [9] , [14] . Together with MD simulations, we address compression mechanisms of these melts and correlate the evolution of structural features with viscosity and density. An atomistic model is established to show that structures of polymerized and depolymerized liquids respond to pressure in distinct manners, resulting in different viscosity and density behaviour. As mobility of silicate melts is primarily controlled by the ratio Δ ρ / η , where η is viscosity of the melt and Δ ρ ( ρ s − ρ m ) is the density contrast between the solid surrounding rock ( ρ s ) and the melt ( ρ m ), the contrasting viscosity and density responses to pressure imply that polymerized and depolymerized melts have rather distinctive dynamic behaviour at depths, thereby profoundly influencing melt transport in deep planetary interiors. Systematics on tetrahedral packing fraction on compression Packing density of liquids increases rapidly with pressure and becomes a key indicator of behaviour and properties at high pressures. In general, less densely packed liquids, such as water and silicates tend to display more complex medium range order (around 3–10 Å), and more abnormal properties, such as negative thermal expansion, than densely packed systems such as liquid metals [32] . Here we examine the tetrahedral packing fraction (TPF) against the measured coordination of normally tetrahedral ions. This packing model is essentially the same as the normalized number density concept presented in ref. 33 , which finds that GeO 2 and SiO 2 glasses increase coordination at the same packing fraction. The present work broadens the concept by accounting for volumes of modifier M (M=Na, Mg, Ca and so on), so that the analysis can be applied to more complex systems. The glass and melt systems examined here include GeO 2 (refs 34 , 35 ), SiO 2 (refs 36 , 37 ), Al 2 O 3 (refs 38 , 39 , 40 ), Al–Si–O (ref. 41 , K/Na/Ca)–Al–Si–O (refs 42 , 43 , Ca/Ba/La/Y)–Al–O (refs 44 , 45 , 46 , 47 , 48 , 49 , Na/Ca/Mg)–Si–O (refs 50 , 51 , 52 , Pb/Nd)–Ga–O (refs 53 , 54 ) and Cs–Ge–O (ref. 55 ) ( Fig. 3 ). The packing fraction of oxygen is described by V O δc O , where V O is the volume of an oxygen atom, δ the atomic number density (in atoms per Å 3 ) and c O the concentration of oxygen in the material. For tetrahedral systems we define V O as the volume occupied by touching spheres of oxygen around the tetrahedrally coordinated cation (see inset of Fig. 3 ). The radius of oxygen atoms ( r O ) is related to the experimentally measured T–O bond length ( r TO ) by r O =(2/3) 1/2 r TO . The presence of network modifiers, whose radii are denoted by r M , occupies additional space. 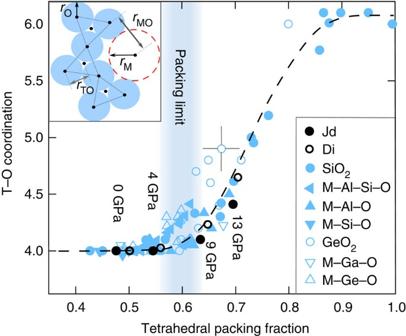Figure 3: T–O coordination versus TPF for a wide range of glasses and melts. The inset illustrates the scheme for TPF calculation: black dots, blue circles and red dashed circles represent sizes of T cations, O and metallic modifiers, respectively. Calculation details are given in the text. Theoretical packing limit, based on hard sphere models, is indicated by the vertical shaded band centred around TPF~0.6. The reported onset of coordination increase is slightly lower than TPF=0.6 in some cases. TPF’s for Jd (solid black circles) and Di (open black circles) melts at various pressures, based on our MD simulations, are also shown, with approximate pressures indicated. At ~4 GPa, average T–O coordination begins to deviate from the value of 4 (tetrahedrally coordinated), signifying the beginning of a network breakup. At ~9 GPa, a significant population of T cations are highly coordinated in both Jd and Di melts. These pressures are based on MD simulations and are slightly different from experimental pressures given inFig. 7. Thus the total TPF of a given melt is Figure 3: T–O coordination versus TPF for a wide range of glasses and melts. The inset illustrates the scheme for TPF calculation: black dots, blue circles and red dashed circles represent sizes of T cations, O and metallic modifiers, respectively. Calculation details are given in the text. Theoretical packing limit, based on hard sphere models, is indicated by the vertical shaded band centred around TPF~0.6. The reported onset of coordination increase is slightly lower than TPF=0.6 in some cases. TPF’s for Jd (solid black circles) and Di (open black circles) melts at various pressures, based on our MD simulations, are also shown, with approximate pressures indicated. At ~4 GPa, average T–O coordination begins to deviate from the value of 4 (tetrahedrally coordinated), signifying the beginning of a network breakup. At ~9 GPa, a significant population of T cations are highly coordinated in both Jd and Di melts. These pressures are based on MD simulations and are slightly different from experimental pressures given in Fig. 7 . Full size image where c M represents the concentration of modifier atoms. In equation (1), the space inside the tetrahedra taken up by Si and Al has been ignored, as the radius of O (~1.38 Å) is much larger than ionic IV coordinated radii of Si (~0.26 Å) and Al (~0.39 Å). Modifier radii are based on the Shannon and Prewitt values [56] and are the largest source of error. Alternatively, r M may be calculated from the measured M–O separation distance minus r O . A single general trend emerges for a wide range of oxide systems ( Fig. 3 ). Below TPF≈0.6, very little coordination increase is observed for both polymerized and depolymerized systems. As TPF approaches 0.6, which roughly corresponds to the packing fraction limit of mono-disperse randomly packed spheres [57] , the coordination begins to increase rapidly. The packing behaviour is most informative at packing fractions below, and close to, the TPF limit (~0.6), where there is essentially zero void space. The tetrahedral network, however, continues to maintain medium range order (3–10 Å), such as ring structures, as modifier ions fill the space between tetrahedra. Above the packing limit, the calculated TPF values no longer reflect realistic packing fractions, as increasing populations of T cations have changed to higher coordination numbers. While the onset of coordination increase occurs at slightly different packing fractions between systems, it is within the errors among the independent measurements. Although some small variation is expected from the different modifier radii, they are within a factor of 1.5 of the oxygen radius, and their concentrations are generally <50% of the oxygen concentration (except for Li, which is an uncommon element in deep earth materials). Within this small variation, the structural evolution of these oxide melts under compression is expected to follow the general trend (the dashed curve, a guide to the eye), regardless of composition or NBO/T ratio. What, then, is responsible for the distinct behaviour in viscosities and compressibilities between polymerized and depolymerized melts? Structural response to compression from X-ray diffraction To examine the contrasting effects of pressure on polymerized and depolymerized silicate melts, we conducted high-pressure synchrotron X-ray diffraction experiments on anhydrous melts along the Jd–Di join, at three compositions Jd, Jd 50 Di 50 and Di, corresponding to NBO/T=0.0, 0.8 and 2.0, respectively. Structure factors S X ( Q ) were obtained from the raw X-ray scattering data using an analytical programme [58] according to the formula, where I X (Q) is the differential X-ray scattering cross-section, I CS (Q) the differential Compton scattering (inelastic) cross-section and f j (Q) the atomic scattering factor of atomic species j , with the summation over all atomic species present in the sample. Q is magnitude of momentum transfer, defined in terms of the scattering angle (2 θ ) and incident X-ray wavelength λ as Q =4 π sin θ / λ . Local structure of the melts in real space is given by the radial (or pair) distribution function, G X ( r ), which is obtained from the Fourier transform where r is the radial distance. More details of the analysis method are given in ref. 59 . Portions of the structure factors S X ( Q ) are shown in Fig. 4a,b . The first sharp diffraction peak (labelled FSDP in the figures) is generally accepted to be related to intermediate-range ordering of the network at separations around 3–10 Å (that is, ~2 π / Q FSDP ), originated from features such as rings of TO 4 tetrahedra [60] . Note that here we use the ‘pre-peak’ definition of FSDP as discussed by Elliot [61] . This definition includes the possibility that the FSDP may be absent (as is the case for most metallic liquids), but for the melts studied here the first peak in the S X ( Q ) is an FSDP, consistent with its structural role, and its broadening and shift to larger Q with increasing pressure. Response of the FSDP position to pressure, measured from the maxima in S X ( Q ), is shown in Fig. 5a —note the consistently decreasing slopes with increasing NBO/T. 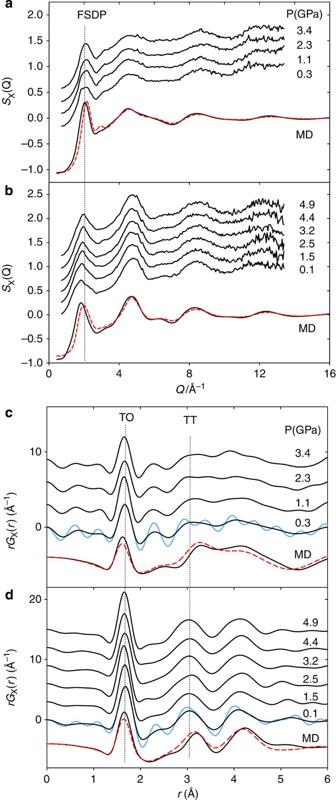Figure 4: Structure factors and deduced partial radial distribution functions. Structure factors and deduced partial radial distribution functionsrGX(r) for Di and Jd melts based on both X-ray diffraction measurements and MD simulations. (a) Structure factors for Di melt. The temperatures at various pressures (with increasing order) are 1,723, 1,873, 1,973 and 2,023 K, respectively. (b) Structure factor for Jd melt. The temperatures at various pressures (with increasing order) are 1,473, 1,623, 1,673, 1,723, 1,873 and 1,923 K, respectively. Estimated temperature uncertainties are about ±50 K. Position of the FSDP is indicated by the vertical dotted line. (c) and (d) showrGX(r)patterns for Di (c) and Jd (d) melts at the corresponding pressures and temperatures. The blue curves, generated using an unmodified transform with aQmax=13.8 Å−1, give an indication of the errors present in the measurements when compared with the black curves, which were generated using a variable modification function, such that the TO peak was not broadened. In each figure, MD simulations at ambient pressure (black solid curve) and 5 GPa (red dashed curve) are shown below the experimental curves for comparison. In (c) and (d), MD lines belowr≈1.2 Å represent the −4πδr2density curve expected at lowr. Figure 4c,d displays variations of G X ( r ) for Di and Jd melts with pressure. The peaks at around 1.6–1.7 Å and 2.9–3.0 Å correspond to the T–O and T–T bond lengths, respectively. The weak peak at ~2.1 Å in Jd melt is a transform artifact owing to the limited Q max and noise present in the measured structure factor. An r -dependent window function was used to discriminate against these transform artifacts [39] , [62] . T–O and T–T bond lengths were determined from G ( r ), and T–O–T angles were calculated using the sine rule and the ratio of these bonds lengths. Figure 4: Structure factors and deduced partial radial distribution functions. Structure factors and deduced partial radial distribution functions rG X ( r ) for Di and Jd melts based on both X-ray diffraction measurements and MD simulations. ( a ) Structure factors for Di melt. The temperatures at various pressures (with increasing order) are 1,723, 1,873, 1,973 and 2,023 K, respectively. ( b ) Structure factor for Jd melt. The temperatures at various pressures (with increasing order) are 1,473, 1,623, 1,673, 1,723, 1,873 and 1,923 K, respectively. Estimated temperature uncertainties are about ±50 K. Position of the FSDP is indicated by the vertical dotted line. ( c ) and ( d ) show rG X (r) patterns for Di ( c ) and Jd ( d ) melts at the corresponding pressures and temperatures. The blue curves, generated using an unmodified transform with a Q max =13.8 Å −1 , give an indication of the errors present in the measurements when compared with the black curves, which were generated using a variable modification function, such that the TO peak was not broadened. In each figure, MD simulations at ambient pressure (black solid curve) and 5 GPa (red dashed curve) are shown below the experimental curves for comparison. In ( c ) and ( d ), MD lines below r ≈1.2 Å represent the −4 πδr 2 density curve expected at low r . 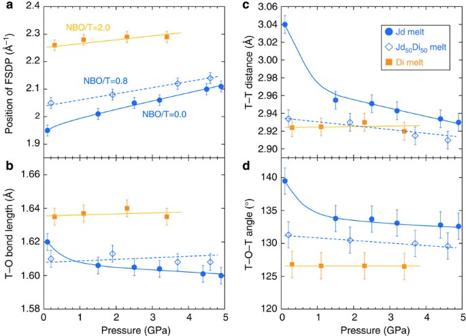Figure 5: Pressure dependence of FSDP and structural parameters for the melts studied. Blue and orange symbols represent polymerized melts (solid circles: Jd, NBO/T=0; open diamonds: Jd50Di50, NBO/T=0.8) and depolymerized melt (solid squares: Di, NBO/T=2), respectively. The curves are a guide to the eye. (a) FSDP as a function of pressure. Note the decreasing slope with an increasing NBO/T ratio in these plots. (b–d) T–O bond length, T–T distance and T–O–T bond angles, respectively. TO4tetrahedra are assumed to remain undistorted within the pressure and temperature range. All four structural parameters show systematic variation with NBO/T. Full size image Figure 5: Pressure dependence of FSDP and structural parameters for the melts studied. Blue and orange symbols represent polymerized melts (solid circles: Jd, NBO/T=0; open diamonds: Jd 50 Di 50 , NBO/T=0.8) and depolymerized melt (solid squares: Di, NBO/T=2), respectively. The curves are a guide to the eye. ( a ) FSDP as a function of pressure. Note the decreasing slope with an increasing NBO/T ratio in these plots. ( b – d ) T–O bond length, T–T distance and T–O–T bond angles, respectively. TO 4 tetrahedra are assumed to remain undistorted within the pressure and temperature range. All four structural parameters show systematic variation with NBO/T. Full size image Figure 5b–d displays three structural parameters: the T–O bond length ( Fig. 5b ), the T–T distance ( Fig. 5c ) and the T–O–T bond angle ( Fig. 5d , calculated from the ratio of Fig. 5b,c ). The fully polymerized Jd melt exhibits clear non-linearity in these structural parameters with increasing pressure. The T–T distance in real space decreases significantly ( Fig. 5c ), whereas the T–O bond length contracts little over the same pressure range ( Fig. 5b ). Assuming that the tetrahedra remain undistorted, these give T–O–T bond angle decreases of 8(2)°, 2(2)° and 0(2)° for Jd, Jd 50 Di 50 and Di melts, respectively ( Fig. 5d ). Structural response to compression from MD simulations MD simulations, fully independent from the measurements, were performed using literature interatomic pair potentials of the form where q α is the charge on atom species α , A and B control the magnitude and decay of the repulsive part of the potential, C controls the magnitude of the van der Waals term and the D term corrects for unphysical attraction at r <1 Å. The unphysical attraction at r <1 Å is a well-known problem for these Buckingham-type potentials, as the r −6 attraction can start to dominate the exponential repulsion. This problem was avoided by including the r −12 term, which is strongly repulsive at low r and negligible for r >1 Å. The constant D αβ was chosen by taking the minimum value that makes the potential and its derivative always positive at low r . Nose–Hoover thermostat and barostats were used [63] ; the time-step was 1 fs. NVT (constant moles, volume, and temperature) simulations were run using the known density of each experimental pressure–temperature point (see Methods for details). Note that for convenience the atomic number density δ (in atoms/Å 3 ) is used. This is related to the mass density ρ (in g cm −3 ) by ρ = δ /0.602214, where A a is the atomic mass of species a and the sum gives the mean atomic weight. S ( Q )s for Jd and Di melts obtained from MD simulations are compared with those determined from X-ray diffraction in Fig. 4a,b , respectively. The corresponding MD radial distribution functions are also given in Fig. 4c,d for comparison. Agreements between X-ray measurements and MD simulations are excellent. 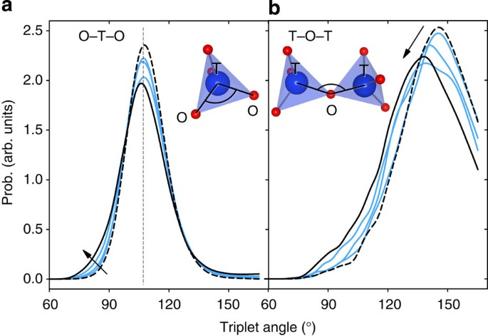Figure 6: Distribution of intra-tetrahedral and inter-tetrahedral bond angle in Jd melt based on MD simulations. (a) The intra-tetrahedral angle O–T–O (see inset for definition) at pressures between 0 GPa (black dashed curve) and 8 GPa (black solid curve), indicating that regular TO4tetrahedra remain the dominant arrangement throughout the pressure range investigated. The small increase at angles <90° (black arrow) is due to an increased population of tri-clusters. (b) Corresponding inter-tetrahedral bond angle T–O–T angle (see inset for definition), showing about 7° shift at ~20% compression (~8 GPa). Blue curves are distributions of T–O–T angles at intermediate pressures. Figure 6a displays the intra-tetrahedral angle within the TO 4 tetrahedron (O–T–O) for Jd melt as a function of pressure. The fact that the angle remains virtually constant within the pressure range of our MD simulations (up to 6 GPa) indicates that TO 4 tetrahedra indeed maintain their regular shape and do not deform significantly, validating the constant inter-tetrahedral angle assumption in deriving Fig. 5d . Similar observations were made on Di melt. The inter-tetrahedral angle (T–O–T) is observed to decrease rapidly with pressure for Jd melt ( Fig. 6b ), consistent with X-ray observations ( Fig. 5d ). Figure 6: Distribution of intra-tetrahedral and inter-tetrahedral bond angle in Jd melt based on MD simulations. ( a ) The intra-tetrahedral angle O–T–O (see inset for definition) at pressures between 0 GPa (black dashed curve) and 8 GPa (black solid curve), indicating that regular TO 4 tetrahedra remain the dominant arrangement throughout the pressure range investigated. The small increase at angles <90° (black arrow) is due to an increased population of tri-clusters. ( b ) Corresponding inter-tetrahedral bond angle T–O–T angle (see inset for definition), showing about 7° shift at ~20% compression (~8 GPa). Blue curves are distributions of T–O–T angles at intermediate pressures. Full size image Detailed accounts of atomic response to compression are summarized in Fig. 7 , where bridging oxygen (BO), NBO and average Si and Al coordination numbers are plotted against pressure. The most striking feature for Jd melt is the monotonically decreasing BO population ( Fig. 7a ) and the increase of oxygen atoms shared by three Al or Si polyhedra (referred to as tri-clusters or TRI– Fig. 7b ). Note that this term is different from ‘tetrahedral tri-clusters’, as not all the polyhedra involved are tetrahedral. Similar observations of triply shared O with various combinations of AlO x polyhedra ( x =4 and 5) have been reported for liquid Al 2 O 3 in ref. 39 . The population of NBO increases slightly, reaching a subtle maximum at a number density of 0.087 atoms/Å 3 , corresponding to ~5 GPa and TPF≈0.57 ( Fig. 3 ). In the absence of TO coordination increase, the transformation of BO into TRI with pressure would most likely be charge-balanced by an increase in NBO population 1/3 the size of the TRI increase. The observed rise in NBO, albeit small and close to the uncertainties of the simulations, is consistent with this expected magnitude. Also, the ambient pressure NBO value deviates slightly from the nominal zero in Jd, owing to a small fraction of these structural features and nano-scale segregation consistent with NMR studies [31] . Overall, average Si–O coordination varies little over the entire pressure range, whereas average Al–O coordination increases with a jump in the slope around TPF≈0.57 ( Figs 3 and 7b ). 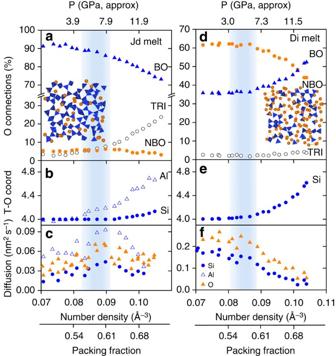Figure 7: MD-simulated structural properties and elemental self-diffusion coefficients (diffusion coefficients in nm2s−1). Left column is for liquid Jd and right column for liquid Di (both at 1,850 °C). For Jd melt, population of BO (solid triangles ina) decreases, even at low pressure, while tri-clusters (open circles ina) and average Al coordination (open triangles inb) increase, with increasing number density or pressure. Population of NBO (orange circles ina) varies little, with a subtle maximum near number density of 0.087 atoms per Å3, coinciding with the kinks in tri-clusters and Al coordination variations (aandb). The average coordination number for Si (solid circles inb) increases very slightly. Self-diffusion coefficients of O (orange triangles), Si (solid circles) and Al (open triangles) all peak at the same pressure (c). For Di melt, initially there is little coordination change. Above about 0.085 Å−3, BO (blue triangles) increases, while NBO (orange circles) decreases (d), and the average Si–O coordination increases (e). Self-diffusion coefficients for O (orange triangles) and Si (blue circles) both decrease monotonically (f). Insets in (a) and (d) are snapshots of the atomic arrangements in Jd and Di melts, respectively. Modifier atoms are shown in orange and tetrahedra are in blue. Figure 7: MD-simulated structural properties and elemental self-diffusion coefficients (diffusion coefficients in nm 2 s −1 ). Left column is for liquid Jd and right column for liquid Di (both at 1,850 °C). For Jd melt, population of BO (solid triangles in a ) decreases, even at low pressure, while tri-clusters (open circles in a ) and average Al coordination (open triangles in b ) increase, with increasing number density or pressure. Population of NBO (orange circles in a ) varies little, with a subtle maximum near number density of 0.087 atoms per Å 3 , coinciding with the kinks in tri-clusters and Al coordination variations ( a and b ). The average coordination number for Si (solid circles in b ) increases very slightly. Self-diffusion coefficients of O (orange triangles), Si (solid circles) and Al (open triangles) all peak at the same pressure ( c ). For Di melt, initially there is little coordination change. Above about 0.085 Å −3 , BO (blue triangles) increases, while NBO (orange circles) decreases ( d ), and the average Si–O coordination increases ( e ). Self-diffusion coefficients for O (orange triangles) and Si (blue circles) both decrease monotonically ( f ). Insets in ( a ) and ( d ) are snapshots of the atomic arrangements in Jd and Di melts, respectively. Modifier atoms are shown in orange and tetrahedra are in blue. Full size image For Di melt, the ratio of NBO/BO also deviates from the nominal 1:1 value ( Fig. 7b ). However, the structural response to pressure is quite different from that of Jd melt: BO increases, rather than decreases, while NBO monotonically decreases ( Fig. 7d ). Average Si–O coordination increases continually ( Fig. 7e ). MD simulations show that O, Si and Al have similar self-diffusion coefficients in Jd and Di melts ( Fig. 7c,f ), supporting the notion that diffusion may involve larger structural units, such as TO 4 [64] . An abnormal pressure dependence with a reversal is also apparent in O, Si and Al diffusivities for Jd melt ( Fig. 7c ). On the basis of the Eyring equation, the reversal in diffusivity with pressure implies a viscosity minimum of around 5 GPa, in broad agreement with experimental results around 2,020 K (3 GPa) (ref. 9 ). For Di melt, however, both Si and O diffusivities decrease monotonically ( Fig. 7f ), implying a monotonic, positive, viscosity response to pressure. The approximate fivefold increase in viscosities up to ~10 GPa, as predicted by the Eyring equation, is in general agreement with investigations using falling-sphere viscometry with in situ high-pressure X-ray imaging [18] , [19] . From the above structural observations, an atomistic picture emerges for the evolution of an anhydrous silicate melt structure under pressure. The structure of polymerized Jd melt may be envisaged as a ‘spongy’ tetrahedral matrix with Na cations ‘stuffed’ into the sponge cavities (inset of Fig. 7a ). Since almost all O anions are BO (NBO/T≈0), the initial response to pressure is to increase the packing fraction by reducing the T–O–T angle ( Figs 3 and 5d ). Because the tetrahedra are heavily interconnected, during initial tightening of the T–O–T angle, some of the BO bonds are broken, weakening the network before any significant T–O coordination increase ( Fig. 7a ). Thus, for Jd melt, and for polymerized melts in general, the initial effect of pressure is to reduce viscosity by ‘depolymerizing’ the structure. With further increase in pressure the TPF limit (≈0.57) is approached ( Fig. 3 ); around this limit coordination begins to increase, along with accelerated formation of tri-clusters ( Fig. 7b ), many of which involving edge sharing of the higher coordinated polyhedra, bringing Jd melt to normal (positive) pressure dependence of viscosity. The role of the more weakly bound Na ions may be viewed as providing internal pressure, through occupying space between the tetrahedra. Na ions may also aid the formation of tri-clusters [65] . Note that above the TPF limit NBO/T is no longer a relevant parameter, owing to the appearance of higher coordinated species, and the relation NBO=2 × O–4T becomes invalid. In Fig. 7 , all the BO and NBO populations are measured based on our MD structural models. Depolymerized Di melt has a much weaker TO 4 network, with ~50% unconnected (NBO) corners at ambient pressure (inset of Fig. 7d ). More closely packed than Jd melt at equivalent number densities (or pressures), Di melt possesses more M–O bonds (M=Ca and Mg) that are considerably weaker than the T–O bonds, providing a ‘cushioning’ mechanism for the TO 4 tetrahedra in compression. Below the TPF limit this weaker structure rearranges without breaking significant amounts of BO bonds or increasing in coordination ( Fig. 7d,e ); decreasing the M–O bond distance is likely the primary mechanism to reduce free volume. Once the packing limit is reached, NBO population decreases rapidly at the expense of BO. This, along with the higher packing fraction, facilitates structural polymerization, hence increasing the viscosity. This atomistic model complements previous thermodynamic treatments on pressure dependence of viscosity of silicate melts [66] . The evolution of BO and NBO with pressure (for example, Fig. 7a,d ) may provide a physical basis for the contribution of polymerization to configurational entropy in the Adam–Gibbs viscosity model [66] . The contrasting effects of pressure on nominally polymerized versus depolymerized melts diminish beyond the TPF limit, above which the structural distinction becomes ambiguous. Thus above TPF≈0.57, NBO/T is no longer relevant for defining the structure and viscosities of silicate melts; all viscosity values fall into a narrower range ( Fig. 1a ) and the general pressure dependence is expected to be positive. Our model also provides insights into the distinct compression behaviours between polymerized and depolymerized silicate liquids. A unique compression mechanism operating in polymerized liquids is the tightening of the T–O–T bond angle ( Fig. 5d ) below the TPF limit. The ‘floppiness’ of the T–O–T angle has significant effects on elasticity of glasses [67] and is likely the cause of low K T0 ′ for polymerized silicate melts. Polymerized melts generally have low densities because they tend to be enriched in Na 2 O, K 2 O, CaO and Al 2 O 3 , and depleted in MgO and FeO. An exception is basaltic melt, which has relatively high FeO contents and low NBO/T, and their density increases more rapidly with pressure owing to low K T0 ′. However, the bond-angle reduction mechanism only occurs at low pressures; with increasing TPF (pressure), the rate of the T–O–T angle reduction decelerates ( Fig. 5d ). Approaching and beyond the packing limit, as populations of higher coordinated species increase and become dominant, this mechanism no longer operates. As a result, K T ′ of polymerized liquids are expected to increase above certain pressure, which likely coincides with the pressure of the viscosity turnover. The above structural effects on viscosity and density of silicate melts have important geophysical implications. Consider basaltic (NBO/T<0.7–0.8) and picritic (NBO/T~0.9) melts in the upper mantle. These polymerized melts reach tetrahedral packing limits typically at around 100–150 km depths [16] , where tetrahedral connections are broken off and higher coordinated Al and Si species begin to form. Major crystalline mantle minerals such as olivine have bulk moduli on the order of 100 GPa, about five times those of the melts, with similar pressure derivatives (K T0 ′≈4; Fig. 2b ). Therefore basaltic and picritic melts are roughly five times more compressible than the solid mantle, before reaching the TPF limit. As the melt ascends (that is, as pressure decreases), the density contrast Δ ρ increases monotonically, providing growing buoyancy that drives magma upwards. Viscosity, on the other hand, varies with pressure by one to two orders in magnitude ( Fig. 1a ), with a minimum at the turnover pressure, greatly reducing flow resistance. The combined effects of pressure and temperature will influence Δ ρ / η drastically from the surface to ~200 km depth. At the depth corresponding to the viscosity turnover, melt mobility (Δ ρ / η ) is expected to reach a maximum. This has been observed for basaltic melt [16] , where melt mobility peaks at around 120 km depth, with Δ ρ / η ~20 times the value near surface and at ~200 km depth, along an adiabatic ascending trajectory. According to the melt zone model [3] , which takes into account the compaction of the solid mantle as the melt migrates [68] , melt volume conservation dictates that melt-filled porosity (that is, melt fraction) varies in a manner proportional to (Δ ρ / η ) −1/2 , while melt velocity is proportional to (Δ ρ / η ) +1/2 , through depth [3] . In other words, where Δ ρ / η is low, melt fraction must be high. Therefore Δ ρ / η plays an important role in controlling magma transport. A better understanding of the distribution of this parameter in depth will help place fundamental constraints on a wide range of long-standing geophysical problems, for example, chemical evolution of early magma oceans and formation of the protocrust [1] , origin of the large igneous provinces [69] , nature of the asthenosphere and the low-velocity zone [16] and magma dynamics of the spreading centres [3] . Sample synthesis Reagent-grade oxides (SiO 2 , MgO and carbonate (CaCO 3 ) for the diopside composition and SiO 2 , Al 2 O 3 and crystalline powder of Na 2 Si 2 O 5 for the jadeite composition, with the latter pre-synthesized from Na 2 CO 3 and SiO 2 ) were mixed in an agate mortar with acetone for 2 h. Each powder mixture was melted at 1,673 K for 5 min. The quenched glasses were crushed and fused again. This process was repeated three times in order to ensure that the glasses were homogenized. Starting material of Di 50 Jd 50 was then prepared by mixing in the diopside and jadeite glasses with 1:1 molar ratio. X-ray diffraction For structure measurements, high-pressure, high-temperature diffraction experiments were carried out using the multi-angle energy-dispersive X-ray diffraction method with a Paris-Edinburgh press (VX3 version) installed at Beamline 16-BM-B of the Advanced Photon Source, in the pressure range of 0.2–4.9 GPa at temperatures from 1,573 to 2,073 K. The cell assembly and pressure and temperature measurement procedure used in this study were identical to that described in ref. 59 . The sample was 2.0 mm in diameter and 2 mm in length, dictated by the maximum achievable pressure. White incident X-rays (5–120 keV) were collimated by vertical and horizontal (0.1 × 0.1 mm) slits made of tungsten carbide (WC). The diffracted beam path was defined by a WC collimator (vertical: 0.1 mm and horizontal: 0.1 mm) and the diffraction signal was collected using a pure Ge solid-state detector with a 4,096 multi-channel analyser, through vertical (5.0 mm) and horizontal (0.1 mm) WC receiving slits. Diffraction patterns were collected at 12 fixed diffraction angles (2 θ =3, 4, 5, 7, 9, 11, 15, 20, 25, 30, 35 and 39.5°) in the horizontal plane. Collection time varied with diffraction angle, as intensities decreased with increasing angles. All patterns were collected until the maximum intensity reached at least 2,000 counts, to ensure reliable counting statistics. The data were analysed using the approach developed in ref. 58 , and the momentum transfer Q in equation (1) was converted from photon energy to wavelength via Q =4 π sin θ / λ =4 πE sin θ / hc , where E , h and c are the photon energies of the polychromatic X-rays, Planck’s constant and the speed of light in vacuum, respectively. MD simulations Classical MD simulations were performed using the DL_POLY classic package. The values of the potential parameters were taken from the work of Du et al. [48] , [50] and Mountjoy et al. [70] ( Table 2 ). The metal–metal interactions, which are not listed, are governed by charge forces only. Table 2 Potential parameters used in the MD simulations. Full size table The simulations of the Jd melt contained a total of ~3,000 atoms, providing a box-size length of 30–34 Å in the pressure-temperature region studied. A similar box size was used for simulating Di melt. The simulations were initiated from a disordered configuration in which the atoms had been moved at random to satisfy a minimum separation distance of 1 Å for all atoms. First a high-temperature NVT (constant volume) run was performed at 6,000 K for 25 ps. The system was then cooled using NPT (variable volume) simulations to 1,300 K for 60 ps, 900 K for 60 ps and 300 K for 120 ps. This resulted in a room temperature glass in which 97.3% of the Al–O and 100% of the Si–O polyhedra were tetrahedral. The final simulated Di and Jd glass densities were within 5% of the measured glass densities. For the self-diffusion, NPT simulations were run at 2,123 K and each temperature–pressure state point was equilibrated for 40 ps before the structure was collected and averaged over the next 100 ps. For the comparison with the X-ray structure factor measurements, the exact temperature and density of the measurements were used in NVT simulations, which were run at 6,000 K for 50 ps, then 3,000 K for 50 ps, before the experimental temperature was run for 100 ps. How to cite this article: Wang, Y. et al. Atomistic insight into viscosity and density of silicate melts under pressure. Nat. Commun. 5:3241 doi: 10.1038/ncomms4241 (2014).